MTCL1 crosslinks and stabilizes non-centrosomal microtubules on the Golgi membrane Recent studies have revealed the presence of a microtubule subpopulation called Golgi-derived microtubules that support Golgi ribbon formation, which is required for maintaining polarized cell migration. CLASPs and AKAP450/CG-NAP are involved in their formation, but the underlying molecular mechanisms remain unclear. Here, we find that the microtubule-crosslinking protein, MTCL1, is recruited to the Golgi membranes through interactions with CLASPs and AKAP450/CG-NAP, and promotes microtubule growth from the Golgi membrane. Correspondingly, MTCL1 knockdown specifically impairs the formation of the stable perinuclear microtubule network to which the Golgi ribbon tethers and extends. Rescue experiments demonstrate that besides its crosslinking activity mediated by the N-terminal microtubule-binding region, the C-terminal microtubule-binding region plays essential roles in these MTCL1 functions through a novel microtubule-stabilizing activity. These results suggest that MTCL1 cooperates with CLASPs and AKAP450/CG-NAP in the formation of the Golgi-derived microtubules, and mediates their development into a stable microtubule network. Microtubules (MTs) are essential for many cellular functions, including vesicle transport, cell motility, polarity and division. These MT-dependent processes are critically dependent on the spatial organization and polarity of MTs, which are controlled by the MT-organizing centre (MTOC). Traditionally, the centrosome has been thought to represent a major MTOC in animal cells [1] . However, many differentiated cells such as polarized epithelial cells and neurons have been shown to develop cell-type-specific arrays of MTs that are not anchored to the centrosome [2] , [3] . Furthermore, recent studies have revealed that, even in less differentiated cells, a subset of MTs is nucleated not from the centrosome, but from the Golgi membrane [4] , [5] , [6] . To date, two groups have independently reported the involvement of two different molecular machineries in this novel nucleation process of MTs. One of the machineries is composed of the MT plus-end tracking proteins, CLASPs, which are anchored to the trans-Golgi membrane via GCC185 (refs 7 , 8 ), and the other is the γ-TuRC (γ-tubulin ring complex)-interacting protein, A-kinase anchoring protein 450 (AKAP450)/centrosome and Golgi localized protein kinase N-associated protein (CG-NAP), which is recruited to the cis-Golgi membrane via GM130 (ref. 9 ). Both machineries have been shown to play critical roles in the development of the Golgi-derived MTs, and thus regulate the formation of the vertebrate-specific higher order structures of the Golgi apparatus. In most vertebrate cells, individual Golgi stacks are laterally connected to form a twisted ribbon-like network, called the Golgi ribbon, which is situated in the juxtanuclear and mostly pericentriolar region of the cell [10] . The maintenance of the Golgi ribbon has been shown to require an intact MT network [11] . However, the underlying mechanism for maintaining this specific Golgi arrangement as well as its physiological significance had been unclear until the above-mentioned studies. They have demonstrated that specific disruption of the Golgi-derived MTs by knockdown of CLASPs or AKAP450/CG-NAP converted the Golgi ribbon into a cluster of Golgi stacks gathering around the centrosome [7] , [9] . Together with data from live imaging analyses [7] , these results have indicated that the formation of the Golgi ribbon proceeds in two distinct steps, in which the Golgi-derived MTs first draw the Golgi ministacks together in a tangential manner, whereas the centrosomal MTs subsequently drag the laterally clustered Golgi stacks towards the centrosome [7] . Interestingly, these studies have also demonstrated that loss of the Golgi ribbon resulted in unpolarized vesicle transport from the Golgi apparatus, and thereby impaired regulated lamellipodia development required for maintenance of directed cell migration [7] , [12] . Taken together, these studies have provided not only new insight into the importance of MTs in organelle architecture, but also evidence for the physiological significance of this vertebrate-specific Golgi architecture. However, in spite of the significant achievements of these studies, the detailed molecular mechanisms underlying the MT nucleation from the Golgi membrane remain to be clarified, although the involvement of γ-tubulin has been demonstrated [8] . In addition, it is unclear how the perinuclear subpopulation of MTs corresponding to the Golgi-derived MTs is specifically stabilized compared with the centrosomal MTs [13] , [14] . We have recently identified a novel MT-regulating protein, MTCL1, which crosslinks MTs through its N-terminal MT-binding region and subsequent coiled-coil motifs, and revealed its indispensable roles in accumulating the non-centrosomal MTs along the lateral membrane of polarized epithelial cells [15] . In the current study, we demonstrate that MTCL1 co-localizes with the Golgi membrane through interactions with CLASPs and AKAP450/CG-NAP, and plays indispensable roles in the development of the Golgi-derived MTs. Correspondingly, MTCL1-depleted cells fail to develop the stable perinuclear MTs and Golgi ribbon. Interestingly, not only the N-terminal MT-binding region, which promotes MT accumulation around the Golgi membrane, but also the C-terminal MT-binding region showing a novel MT-stabilizing activity are required for rescuing these defects in MTCL1-depleted cells. Taken together, the present results suggest that MTCL1 cooperates with CLASPs and AKAP450/CG-NAP for the formation of the Golgi-derived MTs, and mediates their development into a stable Golgi-associated MT network along which the Golgi stacks extend to form the Golgi ribbon. MTCL1 localizes to the perinuclear MTs and Golgi We have previously shown that immunostaining of endogenous MTCL1 in sparsely seeded, less polarized Madin-Darby canine kidney (MDCK) cells revealed granular structures, which intermittently decorated the lateral sides of individual MTs and concentrated at MT bundles [15] . Similar staining was observed in HeLa-K cells ( Fig. 1a ), although enrichment of MTCL1 at one side of the perinuclear region was more conspicuous in these cells. Interestingly, these perinuclear signals of MTCL1 were specifically enhanced when cells were washed with a detergent-containing buffer immediately after methanol fixation ( Supplementary Fig. 1 ). As the enhanced signals disappeared in MTCL1-knockdown cells ( Supplementary Fig. 2 ), these results suggest that MTCL1 epitopes hidden by detergent soluble structures were unmasked by this protocol. Indeed, these perinuclear signals of MTCL1 showed a strong correlation with the distribution of the cis-Golgi marker protein, GM130 ( Fig. 1b ; Supplementary Fig. 2 ). Similar signals were also observed in human retinal pigment epithelial (RPE1) cells ( Supplementary Fig. 2 ). As the Golgi apparatus has an intimate relationship with MTs [11] , these results suggest that MTCL1 may be involved in the regulation of the assembly and/or functions of the Golgi apparatus. 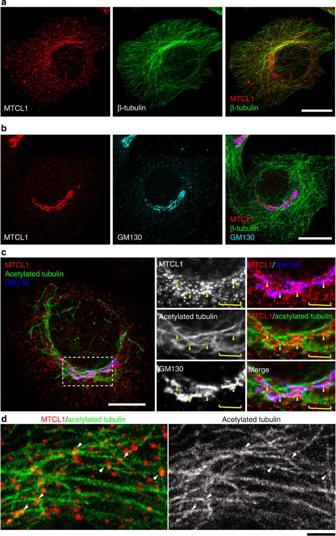Figure 1: MTCL1 localizes to the perinuclear MT bundles associated with the Golgi apparatus. (a) Co-localization of MTCL1 with MTs in HeLa-K cells, which were fixed with cold methanol treatment. Scale bar, 10 μm. (b) Co-localization of MTCL1 with the Golgi apparatus became relatively conspicuous when cells were treated with a detergent-containing buffer immediately after methanol fixation. Note that in comparison withFig. 1a, the signal intensity of MTCL1 was suppressed to optimally visualize the Golgi localization of MTCL1 (see text andSupplementary Fig. 1a). Scale bar, 10 μm. (c) HeLa-K cells were fixed with cold methanol without washing with the detergent-containing buffer and triply stained with MTCL1, GM130 and acetylated MTs. A single confocal plane is shown. Right panels show enlarged views of the boxed region in the left panel. MTCL1 localizes to the contact sites between the Golgi membrane and acetylated MTs (arrowheads). A bracket indicates the region where MTCL1 co-localizes with acetylated MTs, but not with GM130. Scale bar, 10 μm. (d) G-STED super-resolution microscopy revealed the role of MTCL1 in crosslinking the Golgi-associated MTs. The cells were fixed without the detergent wash. MTCL1 and α-tubulin were visualized by Alexa488 and Alexa555, respectively, and super-resolution images were obtained by irradiation with 660-nm STED laser. A single confocal plane is shown. Scale bar, 1 μm. Figure 1: MTCL1 localizes to the perinuclear MT bundles associated with the Golgi apparatus. ( a ) Co-localization of MTCL1 with MTs in HeLa-K cells, which were fixed with cold methanol treatment. Scale bar, 10 μm. ( b ) Co-localization of MTCL1 with the Golgi apparatus became relatively conspicuous when cells were treated with a detergent-containing buffer immediately after methanol fixation. Note that in comparison with Fig. 1a , the signal intensity of MTCL1 was suppressed to optimally visualize the Golgi localization of MTCL1 (see text and Supplementary Fig. 1a ). Scale bar, 10 μm. ( c ) HeLa-K cells were fixed with cold methanol without washing with the detergent-containing buffer and triply stained with MTCL1, GM130 and acetylated MTs. A single confocal plane is shown. Right panels show enlarged views of the boxed region in the left panel. MTCL1 localizes to the contact sites between the Golgi membrane and acetylated MTs (arrowheads). A bracket indicates the region where MTCL1 co-localizes with acetylated MTs, but not with GM130. Scale bar, 10 μm. ( d ) G-STED super-resolution microscopy revealed the role of MTCL1 in crosslinking the Golgi-associated MTs. The cells were fixed without the detergent wash. MTCL1 and α-tubulin were visualized by Alexa488 and Alexa555, respectively, and super-resolution images were obtained by irradiation with 660-nm STED laser. A single confocal plane is shown. Scale bar, 1 μm. Full size image Golgi-associated MTs have been shown to correspond to a specific subset of MTs, which are stabilized and thus rich in acetylated tubulin (see Figs 1c and 2b and Supplementary Fig. 2 ; this subpopulation of MTs is called acetylated MTs, hereafter) [13] , [14] . Therefore, we examined the relationship between the localization of MTCL1, acetylated MTs and the Golgi membranes. When observed in cells fixed without the subsequent detergent wash, many MTCL1 granules were detected at the sites where acetylated MTs made contact with the Golgi membranes (arrowheads). Similar MTCL1 localization was observed in cells at the end of cytokinesis ( Supplementary Fig. 3 ), where MTCL1 not only co-localized with MT bundles accumulated in the midbody, but also localized at the contact sites between the Golgi stacks and the MT bundles emanating from the midbody. These results suggest that MTCL1 has a role in mediating the association of MTs with the Golgi membrane. Moreover, the MTCL1 localization on acetylated MTs, sometimes observed in the regions lacking GM130 signals (a bracket in Fig.1c ), is consistent with its MT-crosslinking activity we have previously demonstrated [15] . Analysis by super-resolution microscopy (G-STED) resolved the perinuclear tracks of acetylated MTs into finer MT strands and revealed that many MTCL1 signals were localized between them or at their intersection points ( Fig. 1d , arrowheads). This is consistent with the results of super-resolution and electron microscopy analyses, demonstrating that the Golgi stacks are embedded in a highly condensed MT network ( Supplementary Fig. 4 ). 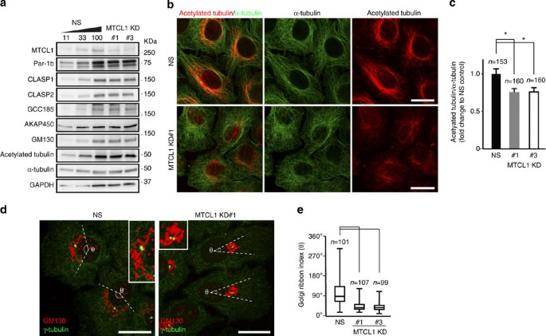Figure 2: MTCL1 knockdown results in reduced accumulation of perinuclear acetylated MTs and disruption of the Golgi ribbon structure. (a) Western blot analysis of MTCL1-knockdown (KD) HeLa-K cells. Cells were transfected with the indicated siRNA oligonucleotides (NS: non-silencing control) and subjected to western blot analysis 48 h later. A threefold serial dilution (11, 33 and 100%) of the non-silencing control sample was loaded as indicated. Note that bothMTCL1siRNAs (#1 and #3) specifically reduced the expression of MTCL1 to <20% of the amount in the control cells without affecting the expression of other proteins involved in Golgi ribbon formation. (b) Effects of MTCL1 knockdown on MT organization. Scale bar, 20 μm. (c) The ratios of immunofluorescence intensities of acetylated tubulin and α-tubulin in (b) were quantified in the projected views generated by simply summing the intensity of each pixel. Data represent the mean±s.e.m. of the indicated number (n) of cells from three independent experiments. *P<0.01, estimated by the two-tailed Mann–WhitneyU-test. (d) Effects of MTCL1 knockdown on the Golgi ribbon structures. Note that the Golgi stacks are clustered around the centrosome stained with γ-tubulin in MTCL1-knockdown cells. Scale bar, 20 μm. (e) Box plot presentation of the Golgi ribbon index corresponding to the laterally expanding angle of the Golgi apparatus around nuclei (θ). The lines within each box represent medians. Data represent the results of the indicated number (n) of cells from three independent experiments. *P<0.01, estimated by the two-tailed Mann–WhitneyU-test. Figure 2: MTCL1 knockdown results in reduced accumulation of perinuclear acetylated MTs and disruption of the Golgi ribbon structure. ( a ) Western blot analysis of MTCL1-knockdown (KD) HeLa-K cells. Cells were transfected with the indicated siRNA oligonucleotides (NS: non-silencing control) and subjected to western blot analysis 48 h later. A threefold serial dilution (11, 33 and 100%) of the non-silencing control sample was loaded as indicated. Note that both MTCL1 siRNAs (#1 and #3) specifically reduced the expression of MTCL1 to <20% of the amount in the control cells without affecting the expression of other proteins involved in Golgi ribbon formation. ( b ) Effects of MTCL1 knockdown on MT organization. Scale bar, 20 μm. ( c ) The ratios of immunofluorescence intensities of acetylated tubulin and α-tubulin in ( b ) were quantified in the projected views generated by simply summing the intensity of each pixel. Data represent the mean±s.e.m. of the indicated number ( n ) of cells from three independent experiments. * P <0.01, estimated by the two-tailed Mann–Whitney U -test. ( d ) Effects of MTCL1 knockdown on the Golgi ribbon structures. Note that the Golgi stacks are clustered around the centrosome stained with γ-tubulin in MTCL1-knockdown cells. Scale bar, 20 μm. ( e ) Box plot presentation of the Golgi ribbon index corresponding to the laterally expanding angle of the Golgi apparatus around nuclei (θ). The lines within each box represent medians. Data represent the results of the indicated number ( n ) of cells from three independent experiments. * P <0.01, estimated by the two-tailed Mann–Whitney U -test. Full size image Effects of MTCL1 knockdown in HeLa-K cells To directly assess the roles of MTCL1 in organizing the Golgi-associated MTs, we examined the effects of MTCL1 knockdown. When MTCL1 expression was specifically reduced in HeLa-K cells to <20% ( Fig. 2a ), the global organization of MTs was slightly disturbed, showing less condensation around the perinuclear region ( Fig. 2b , see the staining of α-tubulin). Far more prominent effects of MTCL1 knockdown were observed with acetylated MTs, which normally showed strong perinuclear condensation around the Golgi apparatus, but exhibited reduced signals and disorganization in MTCL1-knockdown cells ( Fig. 2b and Supplementary Fig. 2 ). Western blot analysis demonstrated that the total amount of acetylated tubulin was not significantly reduced in MTCL1-knockdown cells ( Fig. 2a ). Consistently, the fluorescence intensity of acetylated MTs only revealed 20% reduction in MTCL1-knockdown cells compared with the control cells ( Fig. 2c ). These results suggest that MTCL1 knockdown specifically reduced perinuclearly accumulated acetylated MTs, representing a small subset of the total MTs. When RNAi-resistant MTCL1 was expressed in MTCL1-knockdown cells, the formation of the perinuclear MT bundles rich in acetylated tubulin was restored ( Figs 6c and 7a ). Importantly, ectopically expressed MTCL1 completely co-localized with these MTs, suggesting that the MT-crosslinking activity of MTCL1 mediates the perinuclear accumulation of this subset of MTs ( Figs 6c and 7a ). Figure 6: N-terminal region of MTCL1 is required for the Golgi ribbon formation. ( a ) Schematic illustration of the molecular structure of MTCL1 and its mutants used in the present study. ( b ) The interactions of ectopically expressed V5-tagged MTCL1 wild type or the indicated mutants with endogenous CLASPs and AKAP450/CG-NAP were examined by immunoprecipitation experiments in HEK293T cells. 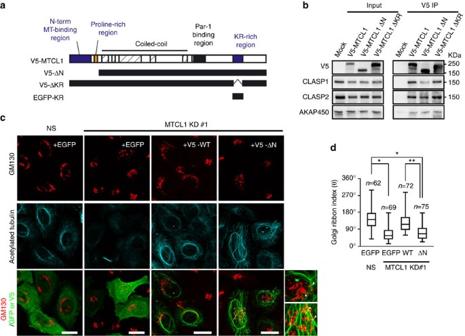Figure 6: N-terminal region of MTCL1 is required for the Golgi ribbon formation. (a) Schematic illustration of the molecular structure of MTCL1 and its mutants used in the present study. (b) The interactions of ectopically expressed V5-tagged MTCL1 wild type or the indicated mutants with endogenous CLASPs and AKAP450/CG-NAP were examined by immunoprecipitation experiments in HEK293T cells. Note that the interactions with both CLASPs and AKAP450/CG-NAP were substantially maintained in the mutants. (c) Rescue experiments demonstrating the importance of the N-terminal region of MTCL1. HeLa-K cells were simultaneously transfected with an expression vector for EGFP, V5-MTCL1 wild type or ΔN, and the indicated siRNA oligonucleotide. After 48 h, they were fixed and stained, to visualize the morphology of the Golgi apparatus (red) and acetylated MTs (cyan). Ectopically expressed proteins were stained with anti-GFP or anti-V5 antibodies (green). Arrowheads indicate the association between the Golgi stacks and the MT bundles induced by V5-MTCL1ΔN. The associations are also indicated in the enlarged views in the small panels on the right. Scale bar, 20 μm. (d) Box plot presentation of the Golgi ribbon index. The lines in each box represent medians. Data represent the results of the indicated number (n) of cells from three independent experiments. *P<0.01 and **P<0.05, estimated by the two-tailed Mann–WhitneyU-test. Note that the interactions with both CLASPs and AKAP450/CG-NAP were substantially maintained in the mutants. ( c ) Rescue experiments demonstrating the importance of the N-terminal region of MTCL1. HeLa-K cells were simultaneously transfected with an expression vector for EGFP, V5-MTCL1 wild type or ΔN, and the indicated siRNA oligonucleotide. After 48 h, they were fixed and stained, to visualize the morphology of the Golgi apparatus (red) and acetylated MTs (cyan). Ectopically expressed proteins were stained with anti-GFP or anti-V5 antibodies (green). Arrowheads indicate the association between the Golgi stacks and the MT bundles induced by V5-MTCL1ΔN. The associations are also indicated in the enlarged views in the small panels on the right. Scale bar, 20 μm. ( d ) Box plot presentation of the Golgi ribbon index. The lines in each box represent medians. Data represent the results of the indicated number ( n ) of cells from three independent experiments. * P <0.01 and ** P <0.05, estimated by the two-tailed Mann–Whitney U -test. Full size image Figure 7: C-terminal KR-rich region of MTCL1 plays a critical role in the Golgi ribbon formation through its MT stabilization activity. ( a ) Rescue experiments demonstrating the importance of the MTCL1 C-terminal region. The experiments were performed as described in the Fig. 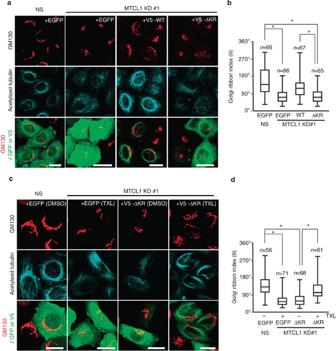Figure 7: C-terminal KR-rich region of MTCL1 plays a critical role in the Golgi ribbon formation through its MT stabilization activity. (a) Rescue experiments demonstrating the importance of the MTCL1 C-terminal region. The experiments were performed as described in theFig. 6c. Note that V5-MTCL1ΔKR could not restore the enrichment of acetylated MTs around the nuclei. Scale bar, 20 μm. (b) Box plot presentation of the Golgi ribbon index in (a). Data represent the results of the indicated number (n) of cells from three independent experiments. *P<0.01, estimated by the two-tailed Mann–WhitneyU-test. (c) Taxol (TXL) compensates for the lack of the KR region for restoring the Golgi ribbon formation. HeLa-K cells simultaneously transfected with an expression vector for EGFP and V5-MTCL1ΔKR were treated with or without 2 μM Taxol for 3 h. Note that when MTCL1-knockdown cells expressed V5-MTCL1ΔKR but not EGFP, they regained the ability to develop perinuclear bundles of acetylated tubulin along with the ability to laterally distribute the Golgi apparatus in response to Taxol treatment. Scale bar, 20 μm. (d) Box plot presentation of the Golgi ribbon index in (c). Data represent the results of the indicated number (n) of cells from three independent experiments. *P<0.01, estimated by the two-tailed Mann–WhitneyU-test. Bar indicates the median. 6c . Note that V5-MTCL1ΔKR could not restore the enrichment of acetylated MTs around the nuclei. Scale bar, 20 μm. ( b ) Box plot presentation of the Golgi ribbon index in ( a ). Data represent the results of the indicated number ( n ) of cells from three independent experiments. * P <0.01, estimated by the two-tailed Mann–Whitney U -test. ( c ) Taxol (TXL) compensates for the lack of the KR region for restoring the Golgi ribbon formation. HeLa-K cells simultaneously transfected with an expression vector for EGFP and V5-MTCL1ΔKR were treated with or without 2 μM Taxol for 3 h. Note that when MTCL1-knockdown cells expressed V5-MTCL1ΔKR but not EGFP, they regained the ability to develop perinuclear bundles of acetylated tubulin along with the ability to laterally distribute the Golgi apparatus in response to Taxol treatment. Scale bar, 20 μm. ( d ) Box plot presentation of the Golgi ribbon index in ( c ). Data represent the results of the indicated number ( n ) of cells from three independent experiments. * P <0.01, estimated by the two-tailed Mann–Whitney U -test. Bar indicates the median. Full size image Recent studies have demonstrated that these perinuclear acetylated MTs correspond to the Golgi-derived MTs, which play essential roles in the lateral connection of the Golgi stacks and inhibit their complete clustering around the centrosome [7] , [9] . Consistent with these reports, MTCL1 knockdown also significantly affected the Golgi apparatus morphology ( Fig. 2d ). In most control cells, the Golgi apparatus formed the ribbon-like morphology in which the Golgi stacks spread broadly in an arc-like manner at one side of the perinuclear region next to the centrosome. In contrast, in MTCL1-knockdown cells, the Golgi apparatus lost its characteristic morphology and showed clustering around the centrosome. Quantitative analysis of the laterally expanding angle (θ) of the Golgi apparatus around the nuclei (Golgi ribbon index) clearly confirmed the effect of MTCL1 knockdown induced by two independent siRNA oligonucleotides ( Fig. 2e ): in control cells, the angle deviated largely depending on the cell cycle stage [16] with a median value of 87.6°, whereas, in MTCL1-knockdown cells, the Golgi ribbon index decreased with a median value of 37.4° and 38.2° for siRNA#1 and #3, respectively. We confirmed that MTCL1-knockdown cells showed a similar cell cycle profile to that of the control cells ( Supplementary Fig. 5 ), indicating that the altered Golgi morphology in MTCL1-knockdown cells was not because of the change in cell cycle progression [16] . These defects were also observed in MTCL-depleted RPE1 cells ( Supplementary Fig. 2 ) and rescued by expression of RNAi-resistant MTCL1 ( Figs 6c and 7a ). Importantly, in the rescued cells, the Golgi stacks regained their expanded distribution along the perinuclear acetylated MT bundles to which ectopically expressed MTCL1 co-localized. Taken together with the results in Fig. 1c , these results indicate that MTCL1 affects the Golgi ribbon formation not only by promoting the perinuclear accumulation of stable MTs, but also by mediating the linkage between the Golgi membrane and MTs. It has been shown that disruption of the Golgi-ribbon structures induced by CLASPs or AKAP450/CG-NAP knockdown resulted in unpolarized cell migration because of defects in polarized vesicle trafficking towards the leading edge [7] , [12] . We also observed similar phenotypes in MTCL1-knockdown cells ( Fig. 3a ). Control cells displayed a classical polarized morphology with a single-dominant lamella at the front and a narrow trailing edge at the rear, and maintained directional migration for several hours ( Fig. 3a ; Supplementary Movie 1 ). In contrast, MTCL1-knockdown cells consistently exhibited a non-polarized morphology with multiple membrane protrusions around the cell periphery during migration ( Fig. 3a ; Supplementary Movie 2 ). As a result, MTCL1-depleted cells showed random migration patterns with reduced directionality of migration ( Fig. 3b,c ). This defect of MTCL1 depletion, which was restored by expression of RNAi-resistant MTCL1 ( Supplementary Fig. 6 ), resulted in retarded wound healing when a monolayer of cells was scratched with a micropipette tip ( Fig. 3d ; Supplementary Movies 3 and 4 ). Interestingly, despite the severe defects in directional migration, MTCL1-knockdown cells still exhibited reduced, but substantial, reorientation of the Golgi apparatus towards the wound compared with the control cells ( Fig. 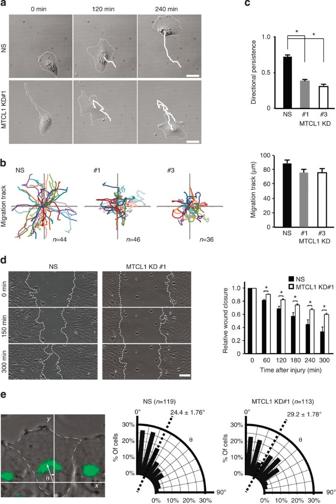3e ). These results may correspond to those observed with AKAP450/CG-NAP-depleted cells [12] and support the notion that not only the Golgi apparatus reorientation, but also Golgi-ribbon formation is crucial for maintaining polarized cell migration [12] . Figure 3: MTCL1 is required for maintaining polarized migration. (a) Typical live imaging data of single RPE1 cells at the indicated time points. Cells transfected with the indicated siRNA oligonucleotide were cultured for 2 days and subjected to live imaging analysis under a differential interference contrast microscope. White dotted lines delineate cell shapes, while white lines show cell trajectories drawn by tracking the centre of the nucleus. Scale bar, 10 μm. (b) Migration tracks (240 min) of cells transfected with the indicated siRNA oligonucleotide.n: total number of the analysed cells from four independent experiments. (c) Top panel: the directional migration of each cell was quantified as the directional persistence defined as the ratio of the direct distance from start to end point divided by the total travel distance during 240 min. Bottom panel: the average travel distances of each cell. Data represent the mean±s.e.m. of the cells analysed in (b). *P<0.01, estimated by the two-tailed Mann-WhitneyU-test. (d) Typical image of wound healing of monolayers of RPE1 cells transfected with the indicated siRNA oligonucleotide. Scale bar, 100 μm. White dotted lines delineate the wound edges. The change in the wound areas was quantified (left). Data represent the mean±s.d. of 15 fields taken from three independent experiments. *P<0.01, estimated by the Student’st-test. (e) The Golgi apparatus polarization towards the wound was estimated as an angle (θ) formed by the cell migration direction (defined as a line perpendicular to the wound) and the lines connecting the nucleus centre and the mass centre of the Golgi ribbon (left panel). Statistically analysed data are presented as radial histograms. The dotted lines represent the mean of angles obtained for the indicated number (n) of cells from three independent experiments. TheP-value estimated by the two-tailed Mann–WhitneyU-test was 0.044 between control and MTCL1-knockdown cells. Figure 3: MTCL1 is required for maintaining polarized migration. ( a ) Typical live imaging data of single RPE1 cells at the indicated time points. Cells transfected with the indicated siRNA oligonucleotide were cultured for 2 days and subjected to live imaging analysis under a differential interference contrast microscope. White dotted lines delineate cell shapes, while white lines show cell trajectories drawn by tracking the centre of the nucleus. Scale bar, 10 μm. ( b ) Migration tracks (240 min) of cells transfected with the indicated siRNA oligonucleotide. n : total number of the analysed cells from four independent experiments. ( c ) Top panel: the directional migration of each cell was quantified as the directional persistence defined as the ratio of the direct distance from start to end point divided by the total travel distance during 240 min. Bottom panel: the average travel distances of each cell. Data represent the mean±s.e.m. of the cells analysed in ( b ). * P <0.01, estimated by the two-tailed Mann-Whitney U -test. ( d ) Typical image of wound healing of monolayers of RPE1 cells transfected with the indicated siRNA oligonucleotide. Scale bar, 100 μm. White dotted lines delineate the wound edges. The change in the wound areas was quantified (left). Data represent the mean±s.d. of 15 fields taken from three independent experiments. * P <0.01, estimated by the Student’s t -test. ( e ) The Golgi apparatus polarization towards the wound was estimated as an angle (θ) formed by the cell migration direction (defined as a line perpendicular to the wound) and the lines connecting the nucleus centre and the mass centre of the Golgi ribbon (left panel). Statistically analysed data are presented as radial histograms. The dotted lines represent the mean of angles obtained for the indicated number ( n ) of cells from three independent experiments. 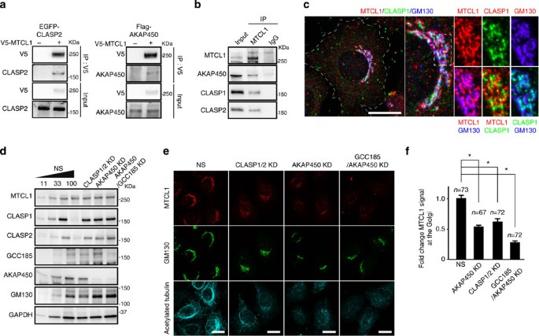The P- value estimated by the two-tailed Mann–Whitney U -test was 0.044 between control and MTCL1-knockdown cells. Full size image Figure 5: MTCL1 is recruited to the Golgi membrane via interactions with the CLASPs complex and the AKAP450/CG-NAP complex. Figure 5: MTCL1 is recruited to the Golgi membrane via interactions with the CLASPs complex and the AKAP450/CG-NAP complex. (a) MTCL1 physically interacts with CLASPs (left) and AKAP450/CG-NAP (right). HEK293T cells were transfected with plasmids expressing EGFP-CLASP2 (left) or Flag-AKAP450/CG-NAP (right) with or without the V5-MTCL1 expression vector. Cell lysates were subjected to immunoprecipitation with V5-antibody, and the immunoprecipitates (IP: V5) were examined with the indicated antibodies. (b) MTCL1 endogenously forms a complex containing CLASPs and/or AKAP450/CG-NAP. RPE1 cells were subjected to immunoprecipitation by an anti-MTCL1 antibody or control IgG (3 μg), and the immunoprecipitates were examined with the indicated antibodies. (c) MTCL1 partially co-localizes with CLASPs as well as GM130 on the Golgi membrane. RPE1 cells fixed with cold methanol and subjected to detergent washing were triple stained with the indicated antibodies. A single confocal plane is shown. Right panels show enlarged images of the boxed region in the middle panel. Scale bar, 20 μm. (d) Western blot analysis of CLASPs and/or AKAP450/CG-NAP-knockdown HeLa-K cells. A threefold serial dilution (11, 33 and 100%) of non-silencing control sample was loaded as indicated. Note that the expression of MTCL1 was not reduced in any knockdown cells compared with the control cells. (e) The Golgi association of MTCL1 depends on both CLASPs and AKAP450/CG-NAP. RPE1 cells were transfected with the indicated siRNA oligonucleotides. After 48 h, the cells were fixed with cold methanol followed by detergent washing, and stained with the indicated antibodies. Scale bar, 20 μm. Note that MTCL1 staining on the Golgi membrane was significantly lower when CLASP1/2 or AKAP450/CG-NAP was depleted. Furthermore, simultaneous knockdown of AKAP450/CG-NAP and GCC185, the Golgi membrane protein anchoring CLASP1 and 2, led to the disappearance of MTCL1 from the Golgi membrane. (f) The ratios of immunofluorescence intensities of MTCL1 and GM130 in (e) were quantified. Data represent the mean±s.e.m. of the indicated number (n) of cells from three independent experiments. *P<0.01, estimated by the two-tailed Mann–WhitneyU-test. ( a ) MTCL1 physically interacts with CLASPs (left) and AKAP450/CG-NAP (right). HEK293T cells were transfected with plasmids expressing EGFP-CLASP2 (left) or Flag-AKAP450/CG-NAP (right) with or without the V5-MTCL1 expression vector. Cell lysates were subjected to immunoprecipitation with V5-antibody, and the immunoprecipitates (IP: V5) were examined with the indicated antibodies. ( b ) MTCL1 endogenously forms a complex containing CLASPs and/or AKAP450/CG-NAP. RPE1 cells were subjected to immunoprecipitation by an anti-MTCL1 antibody or control IgG (3 μg), and the immunoprecipitates were examined with the indicated antibodies. ( c ) MTCL1 partially co-localizes with CLASPs as well as GM130 on the Golgi membrane. RPE1 cells fixed with cold methanol and subjected to detergent washing were triple stained with the indicated antibodies. A single confocal plane is shown. Right panels show enlarged images of the boxed region in the middle panel. Scale bar, 20 μm. ( d ) Western blot analysis of CLASPs and/or AKAP450/CG-NAP-knockdown HeLa-K cells. A threefold serial dilution (11, 33 and 100%) of non-silencing control sample was loaded as indicated. Note that the expression of MTCL1 was not reduced in any knockdown cells compared with the control cells. ( e ) The Golgi association of MTCL1 depends on both CLASPs and AKAP450/CG-NAP. RPE1 cells were transfected with the indicated siRNA oligonucleotides. After 48 h, the cells were fixed with cold methanol followed by detergent washing, and stained with the indicated antibodies. Scale bar, 20 μm. Note that MTCL1 staining on the Golgi membrane was significantly lower when CLASP1/2 or AKAP450/CG-NAP was depleted. Furthermore, simultaneous knockdown of AKAP450/CG-NAP and GCC185, the Golgi membrane protein anchoring CLASP1 and 2, led to the disappearance of MTCL1 from the Golgi membrane. ( f ) The ratios of immunofluorescence intensities of MTCL1 and GM130 in ( e ) were quantified. Data represent the mean±s.e.m. of the indicated number ( n ) of cells from three independent experiments. * P <0.01, estimated by the two-tailed Mann–Whitney U -test. Full size image MTCL1 is essential for the Golgi-derived MTs The above results support the notion that MTCL1 affects the formation of the Golgi-derived MTs similarly to CLASPs and AKAP450/CG-NAP. To directly examine this possibility, we performed nocodazole-washout experiments with RPE1 cells ( Fig. 4 ). As shown previously, complete depolymerization of MTs by nocodazole treatment induced the Golgi fragmentation and dispersion of the Golgi ministacks throughout the cytoplasm ( Fig. 4a left panels, see the staining of the cis-Golgi marker, GS28) [17] . Then, subsequent removal of nocodazole triggered MT regrowth not only from the centrosome, but also from the Golgi ministacks ( Fig. 4a right panels, see the α-tubulin staining) [6] . When the MTCL1 localization was examined in nocodazole-treated RPE1 cells, many MTCL1 signals were still observed on the Golgi ministacks ( Fig. 4a left panels), indicating that MTCL1 interacts with the Golgi membrane independently of MTs. When the cells were subjected to nocodazole washout for 2.5 min, many MT asters radiated from the MTCL1-containing structures on the Golgi ministacks ( Fig. 4a right panels). These results not only support the notion that MTCL1 mediates the linkage between the Golgi membrane and MTs, but also suggest its active involvement in the MT elongation from the Golgi membrane. Indeed, in contrast to the control cells, which developed numerous non-centrosomal MTs within 3 min after nocodazole removal, MTCL1-knockdown cells exhibited markedly low numbers of such MTs ( Fig. 4b,c ). 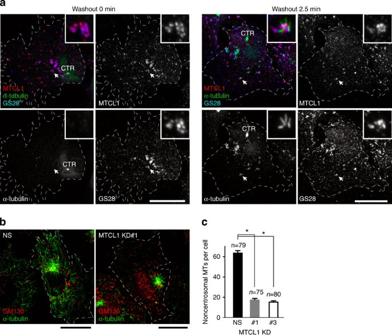We also confirmed a reduction in the Golgi-associated MTs in MTCL1-depleted cells, although a detergent treatment before fixation might disrupt many connections between MTs and the Golgi membrane ( Supplementary Fig. 7 ). These results indicate that MTCL1 plays essential roles in the stable growing of MTs from the Golgi membrane, as has been demonstrated for CLASPs and AKAP450/CG-NAP [8] , [9] . Figure 4: MTCL1 is required for stable development of the Golgi-derived MTs. (a) MTCL1 localization in HeLa-K cells treated with nocodazole. Cells treated with 20 μM nocodazole for 2 h were stained with the indicated antibodies before (left panels) and after (right panels) washing. Note that MTCL1 (red) associated with dispersed Golgi membranes (blue: stained with the cis-Golgi marker, GS28) in the absence of MTs (left panels), whereas MTs (green) grew from the MTCL1-containing structures on the Golgi ministacks immediately after nocodazole washout (right panels). CTR indicates the position of the centrosomes. Scale bar, 20 μm. (b) MTCL1 knockdown reduces non-centrosomal growth of MTs after nocodazole wash. Cells transfected with the indicated siRNA oligonucleotides were cultured for 48 h, and then subjected to the nocodazole washout experiment. The cells were fixed and stained as indicated 2.5 min after nocodazole removal. Scale bar, 10 μm. (c) The number of non-centrosomal MTs in each cell. Data represent the mean±s.e.m. of the indicated number (n) of cells from three independent experiments. *P<0.01, estimated by the two-tailed Mann–WhitneyU-test. Figure 4: MTCL1 is required for stable development of the Golgi-derived MTs. ( a ) MTCL1 localization in HeLa-K cells treated with nocodazole. Cells treated with 20 μM nocodazole for 2 h were stained with the indicated antibodies before (left panels) and after (right panels) washing. Note that MTCL1 (red) associated with dispersed Golgi membranes (blue: stained with the cis-Golgi marker, GS28) in the absence of MTs (left panels), whereas MTs (green) grew from the MTCL1-containing structures on the Golgi ministacks immediately after nocodazole washout (right panels). CTR indicates the position of the centrosomes. Scale bar, 20 μm. ( b ) MTCL1 knockdown reduces non-centrosomal growth of MTs after nocodazole wash. Cells transfected with the indicated siRNA oligonucleotides were cultured for 48 h, and then subjected to the nocodazole washout experiment. The cells were fixed and stained as indicated 2.5 min after nocodazole removal. Scale bar, 10 μm. ( c ) The number of non-centrosomal MTs in each cell. Data represent the mean±s.e.m. of the indicated number ( n ) of cells from three independent experiments. * P <0.01, estimated by the two-tailed Mann–Whitney U -test. Full size image MTCL1 associates with CLASPs and AKAP450/CG-NAP As the above results suggest the possibility that MTCL1 works in cooperation with CLASPs and/or AKAP450/CG-NAP, we examined whether there are physical interactions between these proteins. Figure 5a demonstrates that ectopically expressed V5-tagged MTCL1 specifically co-precipitated with EGFP-tagged CLASP2 or Flag-tagged AKAP450/CG-NAP in HEK293T cells. Furthermore, these proteins were found to interact endogenously, as MTCL1 specifically co-precipitated with CLASPs and AKAP450/CG-NAP from HeLa-K cell extracts ( Fig. 5b ). Previous studies have shown that the CLASPs complex preferentially localizes to the trans-Golgi region [8] , whereas the AKAP450/CG-NAP complex localizes to the cis-Golgi region [9] . Immunofluorescent staining of MTCL1 showed many overlaps not only with the signals of the CLASPs complex, but also with those of the AKAP450/CG-NAP complex (which was identified by an anti-GM130 antibody, because of lack of an appropriate antibody for double staining; Fig. 5c ). These results suggest that MTCL1 interacts with both the CLASPs complex and the AKAP450/CG-NAP complex on the Golgi membrane. Next, we investigated the functional relationship between these proteins. MTCL1 knockdown did not significantly impair the localization of CLASPs and AKAP450/CG-NAP on the Golgi membrane, despite its severe effects on Golgi assembly ( Supplementary Fig. 8a ). Furthermore, immunoprecipitation experiments demonstrated that MTCL1 knockdown did not impair the interaction between CLASPs and GCC185, or between AKAP450/CG-NAP and GM130 ( Supplementary Fig. 8b ), both of which are essential for Golgi membrane association of CLASPs and AKAP450/CG-NAP, respectively [8] , [9] . On the contrary, depletion CLASPs or AKAP450/CG-NAP reduced the localization of MTCL1 on the Golgi membranes ( Fig. 5e,f ) without affecting the expression level of MTCL1 ( Fig. 5d ). It should be noted that depletion of either CLASPs or AKAP450/CG-NAP did not completely abolish the MTCL1 localization on the Golgi membrane. However, simultaneous depletion of AKAP450/CG-NAP and CLASPs (induced by knockdown by GCC185) excluded MTCL1 from the Golgi apparatus more severely ( Fig. 5e,f ). Taken together, these results are consistent with the notion that MTCL1 is recruited to both the trans- and cis-Golgi membranes through binding to the CLASPs complex and the AKAP450/CG-NAP complex, respectively, and cooperates with these machineries to promote stable formation of the Golgi-derived MTs at each site. MTCL1 regulates the Golgi through its effects on MTs As we have reported previously [15] , MTCL1 has two MT-binding domains at the N-terminal and C-terminal regions, the latter termed the KR-rich region (KR; Fig. 6a ). To evaluate whether the MT-binding activity of MTCL1 is essential for its role in regulating the Golgi morphology, we examined the rescue potential of RNAi-resistant MTCL1 (mouse MTCL1) or its mutants lacking either MT-binding domain in MTCL1-depleted HeLa-K cells. First, we examined whether deletion of the N- or C-terminal MT-binding region affects the interaction of MTCL1 with CLASPs or AKAP450/CG-NAP by immunoprecipitation experiments. As shown in Fig. 6b , both mutants retained substantial binding ability to CLASPs and AKAP450/CG-NAP compared with wild-type MTCL1, although the N-terminal deletion slightly reduced the interaction with CLASPs. On the basis of this, we performed rescue experiments by introducing an MTCL1 siRNA oligonucleotide together with an expression vector for EGFP, V5-MTCL1 wild type or its mutants ( Figs 6c and 7a ). EGFP expression did not affect the deleterious effects of MTCL1 knockdown, which disrupted the ribbon-like morphology of the Golgi apparatus and reduced the perinuclear bundles of acetylated MTs ( Fig. 6c,d ). In contrast, as described above, expression of wild-type MTCL1 restored the accumulation of perinuclear MT bundles to which the Golgi stacks were tethered and formed the Golgi ribbon structures ( Fig. 6c,d ). The ΔN mutant (MTCL1ΔN), however, neither restored the normal accumulation of acetylated MTs nor the formation of the Golgi ribbon structures in MTCL1-knockdown cells ( Fig. 6c,d ). It should be noted that probably because of the C-terminal KR-rich region, which can induce MT bundling by itself (see Fig. 8 ) [15] , expression of MTCL1ΔN induced MT bundle formation rich in acetylated tubulin, to which the mutant itself localized. Nevertheless, these MT bundles straggled randomly and did not exhibit complete accumulation around the nucleus. This may be partially because of the reduced binding of MTCL1ΔN to CLASPs, which could cause dissociation of MTCL1ΔN from the Golgi membrane. However, consistent with the substantial association of MTCL1ΔN with CLASPs and AKAP450/CG-NAP ( Fig. 6b ), many Golgi stacks still showed an association with the MTCL1ΔN-induced MT bundles ( Fig. 6c , see enlarged views of the right bottom panel). Therefore, we concluded that the MT crosslinking through the N-terminal MT-binding region also contributes to the normal perinuclear assembly of the Golgi-derived MTs, which are probably required for the Golgi ribbon formation. 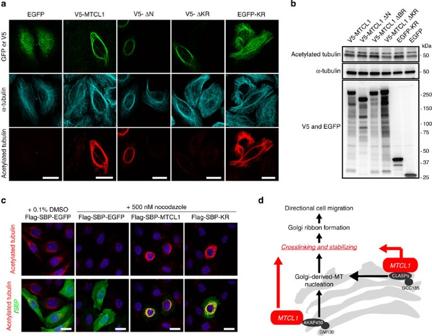Figure 8: KR-rich region has MT stabilization activity. (a) The KR-rich region, but not the N-terminal MT-binding region, is essential for inducing tubulin acetylation in MT bundles. HeLa-K cells were transiently transfected with expression vectors for the indicated proteins. On the next day, cells were fixed and stained to visualize tubulin acetylation as indicated. Scale bar, 20 μm. (b) HEK293T cells were transiently transfected with expression vectors for the indicated proteins at the top. On the next day, total cell extracts were subjected to western blotting to semi-quantitatively assess the increase in tubulin acetylation. (c) HeLa-K cells expressing the indicated proteins were subjected to 500 nM nocodazole treatment for 30 min and examined by immunostaining. Note that the MT bundles induced by wild type Flag-SBP-MTCL1 or Flag-SBP-KR were resistant to the nocodazole treatment. Scale bar, 20 μm. (d) Suggested model for mechanisms through which MTCL1 is involved in the development of the Golgi-derived MTs (see text for detail). Figure 8: KR-rich region has MT stabilization activity. ( a ) The KR-rich region, but not the N-terminal MT-binding region, is essential for inducing tubulin acetylation in MT bundles. HeLa-K cells were transiently transfected with expression vectors for the indicated proteins. On the next day, cells were fixed and stained to visualize tubulin acetylation as indicated. Scale bar, 20 μm. ( b ) HEK293T cells were transiently transfected with expression vectors for the indicated proteins at the top. On the next day, total cell extracts were subjected to western blotting to semi-quantitatively assess the increase in tubulin acetylation. ( c ) HeLa-K cells expressing the indicated proteins were subjected to 500 nM nocodazole treatment for 30 min and examined by immunostaining. Note that the MT bundles induced by wild type Flag-SBP-MTCL1 or Flag-SBP-KR were resistant to the nocodazole treatment. Scale bar, 20 μm. ( d ) Suggested model for mechanisms through which MTCL1 is involved in the development of the Golgi-derived MTs (see text for detail). Full size image Next, we examined the rescue activity of the MTCL1 mutant lacking the C-terminal KR region ( Fig. 7a ). A previous study has demonstrated that this MT-binding region is dispensable for the development of the apicobasal MT bundles in epithelial cells [15] . However, to our surprise, this KR region played a more critical role in the formation of perinuclear MT bundles and the Golgi ribbon than the N-terminal MT-binding region, as, without this domain, MTCL1 could not induce the perinuclear accumulation of acetylated MTs to which the Golgi stacks were tethered. This suggests that the KR-rich region is a prerequisite for stable formation of the perinuclear MT bundles supporting the Golgi ribbon formation. It should also be noted that this mutant was distributed throughout the cells, indicating that the N-terminal MT-crosslinking domain does not function in MT crosslinking without the KR-rich region ( Fig. 8a ). The KR-rich region has MT-stabilizing activity As the KR-rich region resides outside of the central coiled-coil region that mediates MTCL1 oligomerization [15] , this region may indirectly induce MT bundling through its MT-stabilizing activity as has been shown for Taxol and various MT plus-end tracking proteins [18] , [19] . In fact, when overexpressed in HeLa-K cells, the KR-rich region was sufficient to enrich the acetylated tubulin in the MT bundles, which it co-localized with (see EGFP-KR in Fig. 8a,b ). Similar activity was observed with wild type and the MTCL1ΔN mutant, but, interestingly, not with the ΔKR mutant ( Fig. 8a,b ). Furthermore, Fig. 8c demonstrated that the acetylated MTs induced by the KR-rich region corresponded to the stabilized MTs, which showed resistance to nocodazole treatment. Taken together, these results indicate that MTs are stabilized by MTCL1 through the interaction with the C-terminal KR-rich region, but not through the N -terminal region-dependent crosslinking. These results raise the intriguing possibility that the requirement of the KR-rich region for the perinuclear accumulation of acetylated MTs can be attributed to its specific function of stabilizing MTs. If this is true, Taxol may replace the activity of the KR-rich region and compensate for the MTCL1ΔKR defects, to restore the normal accumulation of the acetylated tubulin and the formation of the Golgi ribbon in MTCL1-knockdown cells. As shown in Fig. 7c,d , this is the case. In MTCL1-knockdown cells expressing EGFP, a low concentration of Taxol induced the formation of acetylated MTs, but did not accumulate them around the perinuclear region and restore the Golgi ribbon formation (see +EGFP(TXL) in Fig. 7c ). In contrast, when it was added to the MTCL1-knockdown cells expressing MTCL1ΔKR, Taxol induced significant accumulation of acetylated tubulin around the perinuclear region and, albeit incompletely, made the Golgi apparatus spread out into Golgi ribbon-like structures (see +V5-ΔKR(TXL) in Fig. 7c ). These results demonstrated that one of the critical roles of MTCL1 in the perinuclear accumulation of stable MTs and the Golgi ribbon formation is its MT-stabilization activity mediated by the C-terminal KR-rich region. Previous studies have demonstrated that nucleation of MTs from the Golgi membrane requires CLASPs and AKAP450/CG-NAP [8] , [9] . However, the specific mechanisms by which these proteins promote MT nucleation have not been completely clarified [4] . As enrichment of γ-TuRC on the Golgi membrane compared with the surrounding cytoplasm has not been clearly detected, a ‘selective stabilization model’ has been proposed, in which the Golgi membranes provide the field where unstable MT seeds nucleated from the cytoplasmic γ-TuRC are stabilized for MT elongation [4] . Although a previous study has speculated that the MT plus-end tracking proteins, CLASPs, perform this function by coating the MT seeds [8] , the present study provides an additional and strong candidate for this role, MTCL1, which interacts with the lateral sides of MTs and stabilizes them ( Fig. 8d ). In this study, we demonstrated that the MT-crosslinking protein, MTCL1, preferentially localizes to the perinuclear region, where it associates with not only the Golgi-associated stable MTs, but also with the Golgi membrane. MTCL1 knockdown specifically reduced the perinuclearly accumulated stable MTs and the formation of the Golgi ribbon structure, and both MT-binding regions of MTCL1 were indispensable for rescuing these defects in knockdown cells. Importantly, the C-terminal KR-rich region has MT-stabilizing activity, and addition of a low concentration of Taxol compensated for the lack of this region. In addition, we found that MTCL1 was recruited by CLASPs and AKAP450/CG-NAP to the site where the Golgi-derived MTs nucleate, and played essential roles in MT growth from the Golgi membrane. As ectopically expressed MTCL1 forms significantly stable MTs that cannot be depolymerized with nocodazole, we could not directly examine the involvement of the MT-regulating activity of MTCL1 in the growth of the Golgi-derived MTs. However, the data accumulated in the present work make it highly reasonable to speculate that MTCL1 represents an MT-regulating protein that provides the missing link between CLASPs or AKAP450/CG-NAP and the stable formation of the Golgi-derived MTs ( Fig. 8d ). At the same time, the present results also provide a clear answer to the long-standing mystery of how the Golgi-associated MTs are specifically stabilized [6] . How the cis-Golgi protein, AKAP450/CG-NAP, and the trans-localizing CLASPs can work in concert for this activity [4] is still puzzling, although our results suggest that MTCL1 can support both the AKAP450/CG-NAP-dependent and CLASPs-dependent MT elongation at each site independently ( Fig. 8d ). MTCL1 has been identified as an MT-crosslinking protein in epithelial cells that plays essential roles in accumulating the non-centrosomal MTs into the apicobasal MT bundles [15] . Consistently, the present results suggest that in addition to the MT stabilization activity stated above, MTCL1 functions in accumulating stable MTs around the Golgi apparatus ( Fig. 8d ). In fact, significant MTCL1 staining was observed on the thick MTs associated with the Golgi membrane, and analysis by super-resolution microscopy supported the role of MTCL1 in crosslinking the Golgi-associated MTs. To date, the assembly of the Golgi-associated MTs has not been clearly demonstrated at the ultrastructure level because of the difficulties in preparing optimal specimens to simultaneously reveal longitudinal sections of MTs and the Golgi membranes. In this background, we succeeded to obtain super-resolution images, demonstrating that the Golgi apparatus is embedded in the accumulated, frequently crosslinked, acetylated MTs ( Supplementary Fig. 4a ). This is also supported by our electron microscopy images of HeLa-K cells stably expressing tubulin-copGFP to efficiently identify the region rich in the perinuclear MTs ( Supplementary Fig. 4b ). These results are consistent with the notion that the MT-crosslinking activity of MTCL1 also contributes to the development of the higher order structures of the Golgi apparatus. Importantly, deletion of the N-terminal MT-binding region disturbed the accumulation of the Golgi-associated MTs and the formation of the Golgi ribbon-like structures. This indicates that, as previously observed in epithelial cells [15] , the MT-crosslinking activity of MTCL1 through this domain contributes to the MT accumulation around the Golgi apparatus. As MT bundling induced by the KR-rich region did not cause perinuclear accumulation of MTs ( Fig. 6c ), the flexible crosslinking of MTs through the N-terminal MT-binding region, which is connected to the central coiled-coil region by the proline-rich region ( Fig. 6a ) [15] , may be crucial for the normal function of MTCL1. In this context, it should be noted that the present results provide a sharp contrast to our previous study demonstrating that the KR-rich region is indispensable for the assembly of the non-centrosomal MTs in epithelial cells [15] . Particularly, it is very interesting that, in MTCL1-depleted HeLa-K cells, ectopically expressed MTCL1 could not accumulate MTs when the KR-rich region was missing, even in the presence of the N-terminal region. This indicates that the N-terminal region requires the KR-rich region to interact with MTs. As MTCL1ΔKR could induce MT accumulation in the presence of a low concentration of Taxol, the stabilization of MTs itself, but not the presence of the KR-rich region, appears to be a prerequisite for the N-terminal region of MTCL1 to function. This is consistent with the fact that MTCL1ΔKR can induce MT bundling in wild-type HeLa-K cells, in which endogenous MTCL1 is present and functions in MT stabilization ( Fig. 8a ) [15] . Given that MTs in polarized epithelial cells are stabilized compared with less differentiated cells [20] , [21] , these results further suggest that the N-terminal region may not require the KR-rich region to function in epithelial cells. Recently, the MT minus-end-binding proteins, CAMSAPs, have been reported to exert a strong stabilizing effect on non-centrosomal MTs in epithelial cells [22] , [23] , [24] . They may compensate for the role of the KR-rich region of MTCL1 in these cells. At present, we do not know how the KR-rich region, a sequence of ~100 amino acids showing a high isoelectric point, stabilizes MTs. A similar activity has been observed with the C-terminal MT-binding region of NuMA [25] , [26] , but it shows neither sequence similarity with the KR-rich region of MTCL1 nor enrichment of positive charges. Actually, we could not find regions homologous to the KR-rich region in any other protein. We have already confirmed that the effect of the KR-rich region on MTs does not arise from enhanced acetylation of MTs, as knockdown of Mec-17, which has recently been identified as a critical acetyltransferase of MTs [27] , induced a marked reduction in acetylated MTs in HeLa-K cells, but did not disrupt the Golgi ribbon-like structures ( Supplementary Fig. 9 ). An intriguing idea is that the KR-rich region of MTCL1 stabilizes MTs by binding to the groove between the MT protofilaments, similarly to EB1 and doublecortin [28] , [29] . Detailed analysis of the interaction mode between the KR-rich region and a single-MT strand is required to clarify this issue. In future studies, we also have to substantiate the present hypothesis that the N-terminal region of MTCL1 preferentially interacts with stabilized MTs. Here, we observed that MTCL1-depleted cells showed defects in maintaining polarized cell migration. These results are consistent with the previous studies demonstrating that disruption of the Golgi ribbon and the resultant clustering of Golgi stacks around the centrosome impaired polarized vesicle traffic to the leading edges, causing unpolarized cell migration. We confirmed that wild-type MTCL1, but not either mutant lacking the N- or C-terminal MT-binding region, restored directed migration ( Supplementary Fig. 6 ). These results suggest that at least one of the mechanisms by which MTCL1 contributes to directional migration depends on its positive role in the Golgi ribbon formation through its MT-regulating activity. The additional functions of MTCL1, such as the binding with the cell polarity-regulating kinase, PAR-1, may contribute to this defect of MTCL1-depleted cells, although the PAR-1-binding region is located in the middle of the molecule distal from both MT-binding regions ( Fig. 6a ), and neither the binding with PAR-1 nor the phosphorylation by PAR-1 affects the MT-regulating activity of MTCL1. This issue will be analysed in an independent study that we are currently preparing. In summary, the present study demonstrates that MTCL1 cooperates with CLASPs and AKAP450/CG-NAP for the development of the Golgi-derived MTs through its MT-crosslinking and stabilizing activities ( Fig. 8d ). Considering that non-centrosomal MTs are frequently organized in bundles and are specifically stabilized, these MTCL1 activities may also function in neurons and muscles, in which non-centrosomal MTs are organized in their own specific way. A recent study has demonstrated that the minus-ends of free non-centrosomal MTs present in the cytosol are more stable than previously expected [22] . As MTCL1 knockdown severely affected the non-centrosomal growth of MTs not associated with the Golgi membrane ( Fig. 4 ; Supplementary Fig. 7 ), MTCL1 may also be involved in the stabilization of these cytosolic non-centrosomal MTs in cooperation with MT minus-end-decorating proteins, such as CAMSAPs. Antibodies Anti-PAR-1b and anti-AKAP450/CG-NAP rabbit polyclonal antibodies (pAbs) were generated in house [30] , [31] . Other antibodies were purchased from commercial sources as follows: anti-KIAA0802 pAb and anti-SBP monoclonal antibody (mAb) (SB19-C4) (Santa Cruz Biotechnology); anti-AKAP9 pAb (Novus); anti-CLASP1 and anti-CLASP2 rat mAbs (KT67 and KT68, respectively), anti-GAPDH mAb (6C5) (Abcam); anti-α-tubulin mAb (DM1A), anti-γ-tubulin mAb (GTU-88), anti-acetylated tubulin mAb and anti-GCC2 pAb (Sigma-Aldrich); anti-GCC185 pAb (Bethyl Laboratories); anti-detyrosinated tubulin pAb and anti-β-tubulin mAb (Millipore); anti-GM130 mAb (35/GM130) and anti-GS28 mAb (1/GS28) (BD Biosciences); anti-GFP chicken pAb (Aves Labs); anti-GM130 pAb (MBL); anti-V5 mAb (Life Technologies Corporation). Plasmids V5-tagged mouse MTCL1 and its deletion mutants were subcloned into pCAGGS [32] , pEB6CAG [33] and pEGFP (Takara Bio) [15] . EGFP-KR was constructed using human MTCL1 (KIAA0802) cDNA [15] . For rescue experiments in the cell migration assay, the EGFP was replaced with superfolder GFP (sfGFP) followed by the self-cleaving 2A peptide (P2A) (Life Technologies Corporation). An expression vector for glycosyltransferase (GT)-EGFP (a gift from M. Murata, The University of Tokyo) was used for Golgi visualization [34] . Expression vectors for EGFP-CLSAP2 (a gift from A. Akhmanova, The Utrecht University, The Netherlands) [19] and Flag-AKAP450/CG-NAP [30] were used for co-immunoprecipitation with MTCL1. siRNA oligonucleotides The siRNA oligonucleotide sequences used in this study are as follows: human MTCL1 : 5′-GGUCCAUCUCCGAGAUCGAAG-3′ (#1) and 5′-GGAAUUCUUGUGGAGGAUAGA-3′ (#3); human AKAP450/CG-NAP [9] : 5′-AACUUUGAAGUUAACUAUCAA-3′; human CLASP1 (ref. 35 ): 5′-GGAUGAUUUACAAGACUGG-3′; human CLASP2 (ref. 35 ): 5′-GACAUACAUGGGUCUUAGA-3′; human GCC185 (ref. 36 ): 5′-GGAGUUGGAACAAUCACAU-3′; human Mec17 (ref. 37 ): 5′-ACCGCACCAACTGGCAATTGA-3′ (#2) and 5′-AACCGCCATGTTGTTTATATT-3′ (#3). As a non-silencing RNAi oligonucleotide, All stars negative control siRNA (Qiagen) was used. Cell culture and transfections HeLa-Kyoto (HeLa-K) and HEK293T cells were a generous gift from Dr S. Tsukita (Osaka University, Osaka, Japan) and Dr J. Inoue (The University of Tokyo, Tokyo, Japan), respectively. These cells were cultured in Dulbecco’s modified Eagle medium (DMEM) (Life Technologies Corporation) containing 10% fetal bovine serum, penicillin (100 U ml −1 ), streptomycin (0.1 μg ml −1 ) and 1 mM glutamine at 37 °C in 5% CO 2 . Immortalized human pigment epithelial cells, hTERT-RPE1 (RPE1), obtained from the ATCC were maintained in a 1:1 mixture of DMEM/Ham’s F12 10% fetal bovine serum, penicillin (100 U ml −1 ), streptomycin (0.1 μg ml −1 ), hygromycin B (0.01 mg ml −1 ) and 1 mM glutamine at 37 °C in 5% CO 2 . Plasmid and siRNA oligonucleotide transfections were performed using the electroporation system, NEPA21 (Nepa Gene Co. Ltd.), for HeLa-K cells and RPE1 cells, or Lipofectamine LTX (Life Technologies Corporation) for HEK293T cells, according to the manufacturer’s instructions. To establish GT-EGFP stable transformants, RPE1 cells were transfected with the GT-EGFP expression vector and were cloned through a limiting dilution in 96-well plates in culture medium supplemented with 500 μg ml −1 G418 (Promega). After culturing for 2 weeks, wells containing a single colony were chosen for further study. HeLa-K cells stably expressing tubulin-copGFP were established using a lentivirus vector for the pCT-Tubulin-GFP system (System Biosciences) according to the manufacturer’s instructions. For nocodazole-washout assays, cells were treated with 20 μM nocodazole (Sigma-Aldrich) for 2 h, rinsed five times with ice-cold medium to remove nocodazole, and then allowed to recover in warm (37 °C) medium for appropriate times before fixing and processing for the subsequent immunofluorescence analysis. For the Taxol rescue assay, HeLa-K cells co-transfected with MTCL1 siRNA and the RNAi-resistant rescue constructs were treated with 2 μM Taxol (Sigma-Aldrich) for 3 h before fixing and processing for immunofluorescence analysis. Immunoprecipitation Cells were solubilized in lysis buffer (20 mM Tris-HCl, pH 7.5, 150 mM NaCl, 1% NP-40, 1 mM DTT) containing a cocktail of protease and phosphatase inhibitors (Roche Applied Science) for 30 min at 4 °C, briefly sonicated, and centrifuged at 15,000 × g for 30 min. The resulting supernatants were mixed with Protein G Mag Sepharose (GE Healthcare) conjugated with the appropriate antibodies. To purify V5-MTCL1, anti-V5-tag mAb-conjugated Magnetic beads (MBL) were used. Immunoprecipitates were boiled in SDS sample buffer (10% β-mercaptoethanol, 125 mM Tris–HCl, pH 6.8, 2% SDS, 10% glycerol, 0.005% bromophenol blue) for 5 min and subject to western blot analysis. Western blotting Lysates from HeLa-K cells were extracted with lysis buffer as described above and quantified with the Bicinchoninic acid protein assay kit (Pierce), using bovine serum albumin as standard. Lysates were separated by SDS-PAGE and then transferred to polyvinyldifluoride membranes. Blots were incubated in blocking buffer (5% (w/v) dried skim milk in PBST (8.1 mM Na 2 HPO 4 ·12H 2 O, 1.47 mM KH 2 PO 4 , 137 mM NaCl, 2.7 mM KCl and 0.05% Tween 20)) followed by overnight incubation with the appropriate antibodies diluted in MaxBlot Solution (MBL). Blots were then exposed to horseradish peroxidase (HRP)-conjugated secondary antibodies (GE Healthcare) diluted in blocking buffer for 60 min at room temperature and washed again. Blots were visualized by using the Luminata Forte Western HRP System (Millipore), and chemiluminescence was quantified using the LAS-4000 Luminescent Image Analyzer (FUJI). Full scans of the western blot membranes are provided as Supplementary Fig. 10 . Dilutions of antibodies used were as follows: anti-PAR-1b pAb (1:200), anti-KIAA0802 pAb (1:500), anti-AKAP9 pAb (1:500), anti-CLASP1 rat mAb (1:1,000), CLASP2 rat mAb (1:1,000), anti-GAPDH mAb (1:2,000), anti-α-tubulin mAb (1:2,000), anti-acetylated tubulin mAb (1:2,000), anti-GCC2 pAb (1:200), anti-GCC185 pAb (1:500), anti-detyrosinated tubulin pAb (1:500), anti-GM130 mAb (1:500), anti-GFP chicken pAb (1:1,000), anti-V5 mAb (1:2,000), anti-SBP mAb (1:1,000), and secondary goat anti-mouse, goat anti-rabbit and goat anti-rat HRP-conjugated antibodies (1:2,000). Immunofluorescence HeLa-K cells were seeded on coverslips at a density of 3 × 10 4 cells cm −2 . RPE1 cells were seeded on coverslips coated with fibronectin (50 mg ml −1 , BD Biosciences) at a density of 1 × 10 4 cells cm −2 . To visualize the localization of MTCL1, CLASPs and AKAP450/CG-NAP on the Golgi membrane, cells were fixed with cold methanol for 5 min at −20 °C and rehydrated with PBS containing 0.05% (w/w) Tween 20 for 30 min at room temperature (RT) after a brief wash with the same buffer. When we visualized the localization of MTCL1 on MTs or subjected cells to nocodazole-washout experiments, cells were seeded on coverslips coated with atelocollagen (0.5 mg ml −1 , Koken), fixed with cold methanol for 10 min at −20 °C and washed using PBS without Tween 20. To preserve MT networks or to perform quantitative analysis of assembly structures of the Golgi apparatus, cells were fixed with 4% paraformaldehyde in BRB80 buffer (80 mM PIPES, 1 mM MgCl 2 , 1 mM EGTA, pH 6.8 with KOH) for 5 min at RT, followed by cold methanol fixation (5 min at −20 °C). The fixed cells were pretreated with 10% (v/v) calf serum in TBST (10 mM Tris–HCl, pH 7.5, 150 mM NaCl, 0.01% (v/v) Tween 20) containing 0.1% (w/v) BSA (30 min, RT), and then incubated with primary antibodies diluted in TBST containing 0.1% (w/v) BSA (overnight, 4 °C). Samples were visualized by incubation with the appropriate secondary antibodies conjugated with Alexa Fluor 488, Alexa Fluor 555 or Alexa Fluor 647 (Life Technologies Corporation) (30 min, RT). Dilutions of antibodies used were as follows: anti-AKAP450/CG-NAP pAb (1:300), anti-KIAA0802 pAb (1:500), anti-AKAP9 pAb (1:500), anti-CLASP1 rat mAb (1:200), anti-α-tubulin mAb (1:1,000), anti-γ-tubulin mAb (1:500), anti-acetylated tubulin mAb (1:1,000), anti-β-tubulin mAb (1:1,000), anti-GM130 mAb (1:500), anti-GM130 pAb (1:500), anti-GS28 mAb(1:500), anti-GFP chicken pAb (1:1,000), anti-V5 mAb (1:1,000), and secondary goat anti-mouse, goat anti-rabbit, goat anti-rat and goat anti-chicken Alexa Fluor-conjugated antibodies (1:2,000). Image acquisition and processing Most of the immunofluorescent samples were analysed using the LSM 700 confocal laser scanning microscope (Carl Zeiss Microscopy), equipped with a 63 × 1.4 NA Plan Apochromat or a 100 × 1.46 NA objective. Image files were subsequently processed using the Zen software (Carl Zeiss Microscopy). Unless mentioned otherwise, confocal images are presented as projected views (maximal intensity projection) of several optical sections. To obtain high-resolution images ( Fig. 1c ), the Leica SP8 confocal microscopy system equipped with an HC PL APO CS2 63 × /1.40 oil objective was used in photon-counting mode, and the images were processed using ImageJ software. To obtain super-resolution images ( Fig. 1d ), samples mounted in Prolong Gold (Invitrogen) were observed using a Leica TCS SP 8 Gated Stimulated Emission Depletion (G-STED) microscope (Leica) equipped with an HC PL APO CS2 100 × /1.40 oil objective. Samples visualized with Alexa488 and Alexa555 were irradiated with 660 nm STED laser, and the G-STED parameters were optimized for best resolution. The laterally expanding angle of the Golgi apparatus around nuclei was quantified using the ImageJ plug-in ‘Measure’. Differential interference contrast (DIC) images were obtained using a DM IRE2 inverted microscope (Leica Microsystems) equipped with an HC PL Fluor × 20/0.5 objective. Cell migration tracks were quantified with the ImageJ plug-in ‘Manual tracking’ by tracing the centre of each cell in the DIC recordings of migrating single cells as reference points. In rescue experiments, cells expressing RNAi-resistant MTCL1 were identified by fluorescent signal of co-expressing sfGFP. Directional persistence was quantified as the final distance of cell relocation divided by the total migration track. For the wound-healing assay, RPE1 cells stably expressing GT-EGFP were transfected with control or MTCL1 siRNAs and plated on glass bottom culture dishes (MatTek). Two days later, wounds were made by scratching cell monolayers with a micropipette tip. Fluorescent images of cytosolic sfGFP (separated from MTCL1 by the endogenous cleavage in the 2A peptide sequence), GT-EGFP and phase contrast images were obtained using a Biostation CT equipped with Plan Fluro ADL × 10 objective (Nikon), and processed using CL-Quant with the wound-healing analysis procedure (Nikon). Golgi apparatus polarization was estimated as an angle (θ) formed by the cell migration direction (defined as a line perpendicular to the wound line) and the lines connecting the nucleus centre and the mass centre of the Golgi ribbon-like structures (see Fig. 3e , left panel). Transmission electron microscopy Transmission electron microscopy was performed in essentially the same manner as described elsewhere [38] . In brief, HeLa-K cells cultured on coverslips were fixed with 2% fresh formaldehyde and 2.5% glutaraldehyde in 0.1 M sodium cacodylate buffer, pH 7.4, for 2 h at RT. After washing with 0.1 M cacodylate buffer, pH 7.4, they were postfixed with ice-cold 1% OsO 4 in the same buffer for 2 h. The samples were rinsed with distilled water, stained with 0.5% aqueous uranyl acetate for 2 h or overnight at RT, dehydrated with ethanol and propylene oxide, and embedded with an embedding kit (Poly/Bed 812; PolySciences). After removal of the coverslips using ice-cold hydrofluoric acid, ultra thin sections were cut, doubly stained with uranyl acetate and Reynolds’ lead citrate, and viewed with a transmission electron microscope (JEM-1010; JEOL) with a charge-coupled device camera (BioScan model 792; Gatan) at an accelerating voltage of 100 kV. To efficiently identify optimal fields for perinuclear MT observation, we used HeLa-K cells stably expressing tubulin-copGFP seeded on coverslips with a numbered grid (150-μm grid; Matsunami Glass Industry) , and observed them under fluorescent microscopy before the electron microscopy analysis. Fluorescence-activated cell sorting Cell cycle profiles were analysed in HeLa-K cells (1 × 10 4 cells) on a FACS Canto II flow cytometer (BD Biosciences) by MODFIT LT ver. 2.0 software. In brief, cells were washed once in PBS and fixed in 70% ethanol. After washing with PBS, cells were incubated in PBS containing 50 μg ml −1 propidium iodide (Life Technologies Corporation) and 0.625 mg ml −1 DNase-free RNase (Qiagen) for 30 min at room temperature in the dark and then analysed for propidium iodide fluorescence intensity. How to cite this article: Sato, Y. et al. MTCL1 crosslinks and stabilizes non-centrosomal microtubules on the Golgi membrane. Nat. Commun. 5:5266 doi: 10.1038/ncomms6266 (2014).